Structured patterns in geographic variability of metabolic phenotypes inArabidopsis thaliana Understanding molecular factors determining local adaptation is a key challenge, particularly relevant for plants, which are sessile organisms coping with a continuously fluctuating environment. Here we introduce a rigorous network-based approach for investigating the relation between geographic location of accessions and heterogeneous molecular phenotypes. We demonstrate for Arabidopsis accessions that not only genotypic variability but also flowering and metabolic phenotypes show a robust pattern of isolation-by-distance. Our approach opens new avenues to investigate relations between geographic origin and heterogeneous molecular phenotypes, like metabolite profiles, which can easily be obtained in species where genome data is not yet available. The naturally occurring accessions of Arabidopsis thaliana (Arabidopsis) are found across continents and have adapted to various growth habitats [1] , [2] , [3] . This together with their known genetic basis and geographic origin has led not only to the identification of ecologically relevant traits [4] , [5] , [6] , [7] , but also global patterns of genetic diversity [8] , [9] , [10] and their relation to climate [11] , [12] . Recently it was discovered that genetically similar Arabidopsis accessions derive from geographically more closely related locations, suggesting a robust pattern of isolation by distance [13] , [14] , [15] . However, these findings were obtained by relating the genetic and geographic distances either across all accession pairs or via parameter-dependent neighbourhood structures, and without correcting for climate effects. They were also restricted to genotypic variation, whereas selection will act on phenotypic traits. Here we provide a parameter-free network-based approach for mapping heterogeneous molecular phenotypes on networks constructed from geographic location data. We use this approach in combination with corrections for climate effects to demonstrate that not only genotypic variability, but also flowering and metabolic phenotypes robustly relate to geographic origin of Arabidopsis accessions as predicted by the isolation-by-distance model. Phenotypic and genotypic data sets Metabolic profiles contain information about the levels of large numbers of metabolites. They provide an integrative phenotype that has already been shown to be predictive of biomass yield [16] , [17] , [18] , heterosis [19] and, to a lesser extent, abiotic stress tolerance [20] , as well as to be indicative of wine quality from different sites [21] , [22] , [23] . We analysed the levels of 49 metabolites in 92 diverse accessions, including lines with different growth habitats and geographic origins ( Supplementary Table S1 ). The majority of the analysed accessions come from Eurasia, together with a few accessions from North America and Africa. The accessions were grown ex situ under standardized irradiance, photoperiod and temperature. Metabolic profiles were determined in a 12-h light/12-h dark photoperiod at two levels of nitrogen fertilization: one allowing close to maximal growth (OpN) and another limiting growth (LiN) [24] , as well as in a 8-h light/16-h dark photoperiod with high nitrogen supply when growth is limited by carbon (LiC) [25] . Carbon is the major component of plant biomass, and short photoperiods lead to a coordinated decrease in metabolism and growth to maintain a balance between photosynthetic assimilation, storage and use of carbon [26] , [27] . Nitrogen is often a limiting nutrient of plant growth, and the molecular basis for its assimilation by plants is well-established [28] . Uptake and remobilization of nitrogen have been investigated in a small number of Arabidopsis accessions [29] , [30] , [31] , [32] , [33] , but the extent to which variation in metabolic processes reflect adaptations to specific environments and how this variation is maintained with regard to geographic proximity and climate remain elusive. As further data sets, we used a publically available data set for flowering phenotypes covering 40 of the 92 accessions [34] , and two independent single-nucleotide polymorphism (SNP) data sets [13] , [15] covering 69 and 80 of the 92 accessions, respectively ( Supplementary Table S2 ). Analysis based on dense structure To gain insight into dependence on geographic origin, we first generated distance matrices for genotype and for each phenotype, as well as for geographic locations. The resulting matrices retain information about the relationships between all pairs of accessions, and, thus, are representative of the dense or global structure. The relation between the matrices was examined with the help of the Mantel correlation [35] ( Supplementary Fig. S1 ). 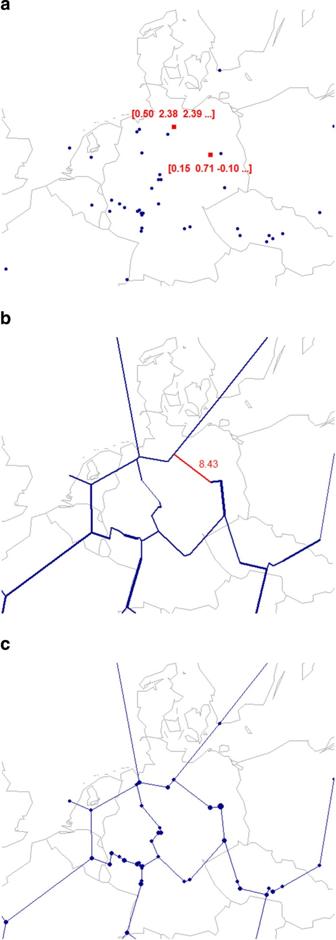Figure 1: Mapping of molecular profiles on proximity networks. (a) Location of the Central European lines (blue) together with illustration of metabolic profiles for two accession lines (red); (b) RN network on the Central European lines including edge-weight—the Euclidean distance of the profiles of the highlighted accessions (red); (c) Geographic distribution ofon the RN network in Central Europe when metabolic profiles are used. The size of a circle corresponds to the corresponding value of. The analysis indicated that the Mantel correlation between geographic and genomic distance is positive and significant at level 0.05 ( Table 1 ). Analogous analysis of the relation between the difference in flowering phenotypes and geographic distances suggest smaller and non-significant correlation values. For the OpN metabolic phenotype, positive and significant correlation was observed. This indicated that in near-optimal growth conditions, differences in metabolite profiles, like those of SNPs, become larger with increased spatial dispersion, thus hinting at isolation by distance. This relation broke down for metabolite profiles collected in carbon-limited plants and nitrogen-limited plants, for which a non-significant positive relation and a slightly negative relation was found, respectively. Table 1 Results from analysis on dense structure. Full size table To exclude the effect of climate from these analyses, we calculated the partial Mantel correlation between differences in genotype or phenotypic trait and geographic distances while controlling for the following five climate variables: daily minimum, average, and maximum air temperatures, relative humidity and daylight hours [36] . When the effect of climate is controlled, the partial Mantel correlation between geographic and genomic distances was positive and smaller than for the full correlation, but not always significant ( Table 1 ). We did not find a significant correlation either between the geographic distances and differences in flowering phenotypes or between geographic distances and differences in OpN, LiN or LiC metabolic phenotypes, although the OpN and LiC remain positive while LiN is negative. This indicates that relationships found in the analysis of the dense structure may be at least partly driven by climatic factors, which will recur at different places on the globe, rather than geographical distance per se. Sparse network-based approach for local structure We next investigated whether there is a consistent relation between differences in proximity structure of accessions and genotype or phenotypic traits. Proximity structure captures the sparse or local geographic relations between accessions, and is given by the relative neighbourhood (RN) network [37] ( Fig. 1a ). The RN network provides a well-defined reference for mapping of various phenotypic data. It was generated from bilateral relationships, whereby two accessions are considered neighbours if there is no other accession at a smaller geometric distance. The distance between the phenotype, p , of two adjacent accessions (that is, nodes) was used to calculate the weight of the corresponding edge ( Fig. 1b ). Each node u is in turn described by , the average of the edge-weights incident on it ( Fig. 1c ). The entire network G is characterized by , the average of the resulting node-weights. The lower the value of , the more similar the metabolic phenotypes between neighbouring accessions. The salient network properties of the networks resulting from the three conditions are summarized in Supplementary Table S3 . We note that with this approach, geographic distances were considered in setting up the RN network, but not in weighting of the nodes and edges. This renders the approach free of subjectively imposed distance cutoffs. Figure 1: Mapping of molecular profiles on proximity networks. ( a ) Location of the Central European lines (blue) together with illustration of metabolic profiles for two accession lines (red); ( b ) RN network on the Central European lines including edge-weight—the Euclidean distance of the profiles of the highlighted accessions (red); ( c ) Geographic distribution of on the RN network in Central Europe when metabolic profiles are used. The size of a circle corresponds to the corresponding value of . Full size image Geographical origin analysis based on sparse structure The weighted RN network was used to investigate the pattern of local changes in respect to geographic origin. The relationship between proximity structure and genotype or phenotype was explored by using three statistics from classical geographic variability (GV) analysis, namely: Moran’s I [38] , Geary’s C [39] , and the Global G [40] . The first two statistics test the hypothesis that there is spatial relationship between quantities mapped on the network with the null hypothesis of homogeneous spatial distribution. Global G statistic tests whether there are spatial bursts of high (or low) values in an otherwise homogeneous space. 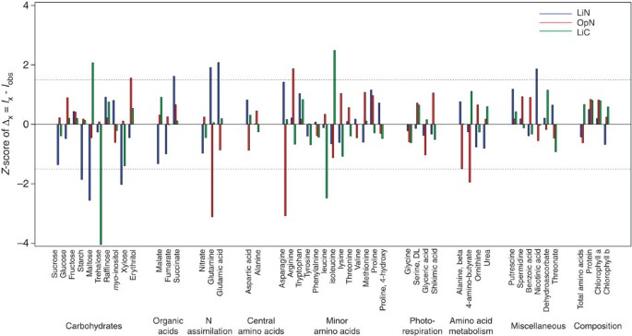Figure 2: Most influential metabolites for the considered accessions. The distribution of the absolute values of thez-scores foris depicted for LiN, OpN and LiC conditions. Negativez-scores are shown with hatch-marks. The metabolites whose absolute values ofz-scores are at least one and a half s.d.’s above the mean (shown by a dashed grey line) are considered to have the highest effect on the GV analysis. All three statistics indicated positive relations of flowering phenotypes and the three metabolic phenotypes with geographic distance ( Table 2 ). However, with these accessions ( Supplementary Table S2 ), we did not observe an isolation-by-distance model for genotypic differences; Moran’s I and Geary's C statistics based on indicated the absence of statistically significant positive relation between genotypic differences of neighbouring accessions ( Table 2 ). These findings suggest that metabolic and flowering phenotypes are likely to show highly convergent local adaptation following the isolation-by-distance model even when neighbouring accessions may exhibit larger genetic variation. Table 2 Results from analysis based on weighted RN network. Full size table In addition, we considered whether the metabolite profiles might be related to flowering traits, which would mean that these two phenotypes are not truly independent. The plants used for the metabolomics analysis were harvested long before floral induction. Analysis of the correlation structure between the metabolite and flowering phenotypes across 40 accessions ( Supplementary Fig. S2 , Supplementary Table S4 ) demonstrated the lack of a consistent relationship across the three conditions. This was further supported by the lack of congruence for pairs of the resulting correlation matrices across conditions, as demonstrated by the RV coefficient ( Supplementary Table S5 ), suggesting a complex interplay between the two phenotypes [41] . Taken together, when sparse analysis was used, isolation-by-distance was observed at the level of metabolic and flowering phenotypes but not at the level of genetic variability for the analysed accessions ( Supplementary Table S2 ). The absence of a relationship with genotypic distance apparently contrasts with recent studies, which reported isolation by distance [13] . Nevertheless, performing the proposed analysis by using the RN network on a larger set of 170 accessions [34] indicated that isolation-by-distance model was also confirmed with SNP data ( Supplementary Table S6 ). Moreover, the values for the statistics were in quantitative agreement with those obtained from metabolic and flowering phenotypes ( Table 2 and Supplementary Table S6 ). This raises the question why isolation-by-distance at the level of genetic variability is only revealed when the sparse analysis is performed with a larger number of accessions. As recent studies [42] , [43] have demonstrated that only 9.4–18.5% of SNPs in A. thaliana are functionally relevant, the usage of the whole set of SNPs may introduce artifacts and reduce the robustness of the statistics, particularly pronounced in smaller populations (as demonstrated in the analysis of robustness). Moreover, whole-genome scale SNP variation also includes neutral variation, which may mask the genetic patterns that are solely due to local adaptation, especially with limited number of accessions, whereas metabolic and flowering traits are more likely directly under natural selection. The proposed mapping of heterogeneous phenotypes on the RN network used in our sparse analysis can reduce bias in examining differences in phenotypes, as it does not consider relations between otherwise unrelated accessions generated from the k nearest neighbours ( k NN) of each accession [13] . In contrast to the k NN network, which may include unilateral relationships and is dependent on the arbitrarily chosen parameter k , the RN network is not only more stringent but also uniquely determined by the locations of the analysed accessions. To emphasize this claim, we compared the results from the RN and k NN network ( Supplementary Table S7 ): examination of the three statistics based on the k NN network demonstrated that their values change drastically with varying k . This implies that a sound conclusion in support of the isolation-by-distance model cannot be readily obtained with the k NN network as there is no objective rule for the selection of a value for k . Metabolites related to pattern formation To determine whether a particular metabolite has an effect on the autoregressive model for , we calculated the difference in the Moran’s I statistic from the metabolic phenotypes with and without the metabolite. Metabolites are then ranked based on the z -normalized differences, which separates two classes of opposite effect. The z -scores across all metabolites are presented in Fig. 2 . In LiN, carbohydrates and amino acids had opposite effects, with negative values for many carbohydrates like starch, maltose and xylose, and positive effects for central amino acids like glutamine and glutamate, as well as nicotinic acid. The presence of carbohydrates and nitrogen containing metabolites points to metabolism in nitrogen limiting condition as a single yet tightly connected large network [44] . The pattern was strikingly different for the OpN phenotype, with very strong negative values from the two nitrogen-rich amino acids, glutamine and asparagine, and smaller values from β-alanine and 4-amino-butyric acid, two intermediates in amino acid degradation. In LiC, there is a strong effect for maltose, trehalose, leucine and isoleucine. Figure 2: Most influential metabolites for the considered accessions. The distribution of the absolute values of the z -scores for is depicted for LiN, OpN and LiC conditions. Negative z -scores are shown with hatch-marks. The metabolites whose absolute values of z -scores are at least one and a half s.d.’s above the mean (shown by a dashed grey line) are considered to have the highest effect on the GV analysis. Full size image Robustness of findings To investigate the robustness of the statistics from the analyses of dense and sparse structures, we repeated the analysis following exclusion of 5–25% of the analysed accessions. Our findings indicated a general trend that the variability of the statistics on the sparse structure, captured in the RN network together with the proposed mapping of phenotypes, was smaller than the variability of the statistics on the dense structure. In addition, consistently smaller variability was found for the statistics based on the metabolic phenotype than for genomic data, as indicated by the values of the squared coefficient of variation ( Table 3 ). To capture the effects of the sparse proximity structure in combination with climate factors, we also tested a spatial simultaneous autoregressive model for . The spatial parameter is positively significant, with a value of 0.66, 0.81 and 0.75 for the metabolic phenotypes under OpN, LiN and LiC conditions, respectively. None of the other factors significantly influences the regression ( Supplementary Table S8 ). Table 3 Robustness of statistics from analyses based on dense and sparse neighbourhood structure. Full size table To summarize, our results show that patterns of ecological isolation can be robustly identified with the proposed method for mapping genotypic variation and metabolic and flowering phenotypes on sparse proximity structure. This approach avoids potential inclusion of bias due to heterogeneity of geographic terrain, which often implies usage of air distances and various distance-related cutoffs. Moreover, we demonstrate that the three statistics commonly used in GV analysis reveal the congruence between two very different phenotypic traits: flowering phenotypes and metabolic phenotypes. This opens up the possibility of a research strategy for analysing proximity relations in less well-characterized species for which genome data is not yet available, including closely related species whose genomes are divergent enough to require de novo assembly, but for which metabolic phenotypes would be facile to obtain. Distance measures The different types of data require specific distance measures to investigate how phenotypic and genetic variability relate to geographic origin. To facilitate approximations of Euclidean distances due to Earth curvature, the longitude and latitude are converted from radial units to kilometres by multiplying the given figures with 53 and 69.1 km, respectively. To reduce artifacts, the remaining types of numeric profiles are first z -normalized. Distances between z -normalized numerical profiles are obtained based on the Euclidean metric. Distances between DNA fingerprints [13] and SNP data [15] , [34] are determined by a simple count of pair mismatches. While DNA fingerprints warrant the usage of modified scores, following probabilistic treatment of wildcards, for reasons of objective comparison between the two data sets on genetic variability we did not further consider this approach. Analysis based on dense global structure To determine how phenotypic variability and genetic diversity relate to geographic location, the distance measures detailed above were applied to each profile type across all pairs of accessions. The resulting distance matrices capturing all-to-all accession differences were analysed by using the Mantel correlation as implemented in the function mantel from the ecodist package in R [45] ( Supplementary Fig. S1 ). To exclude the effect of climate, we determined the partial Mantel correlation while controlling for the five climate characteristics enumerated above. The calculations for the partial Mantel correlation were performed by using the same function in R. Analysis based on sparse local structure GV analysis seeks to identify patterns of genotypic or phenotypic relatedness dependent on the geographic positions and patterns of dispersal for biological entity of interest. To this end, one or more variables are commonly mapped onto a set of given geographic sites, specified by their respective longitude and latitude, or areal unit centroids (see ref. 46 and references therein). While in the classical GV analyses, these variables may be interval, ordinal, or nominal, with the advances in high-throughput technologies, biological entities are often described by vector profiles including different system level responses (for example, transcriptomic, proteomic, metabolomic) to genetic and/or environmental perturbations. Many of the techniques from GV analysis require specification of the geographic proximity between the entities which, in turn, can be employed to establish the adjacency relations. The pattern of geographic variation of a variable of interest can then be evaluated with regard to the interconnectedness of the sampling location for which the variable has been measured or observed. To discern such patterns, one usually uses various statistics determining how the variable’s level for each entity is correlated with an appropriately scaled average of the levels from the entity’s neighbours. As the correlation is calculated on the same variable, it is usually referred to as spatial autocorrelation. The correlation can be global, as in the case of the Moran’s I statistics [38] , which assumes spatial homogeneity, or can take into account local effects, such as the case of the Geary’s C statistics [39] and Anselin’s local indicators of spatial association [47] . Therefore, it is obvious that any analysis of the spatial autocorrelation in the case when each biological entity is described by its location and is attributed a variable in a vector form requires: ( i ) an appropriate choice of the definition for geographic proximity and ( ii ) a novel statistical method which can be used in identifying the patterns with such variables. RN network Geometric networks provide a formal way to capture the concept of proximity (referred to as neighbourhood) often encountered with geographic locations specified by their longitude and latitude. In geometric networks, the nodes describe the spatial (geographic) locations of given entities (nodes), and two nodes are connected by an edge if a well-defined neighbourhood is empty. The neighbourhood is called empty if and only if no location lies in its interior (except when entire half-space is involved). Let d ( x , y ) denote the distance between any two nodes x , y S . In all calculations, we consider the Euclidean distance between the two nodes, that is, . In the following, we consider the RN network, whereby two nodes x and y from a given set of nodes S are defined to be adjacent (that is, proximal) if and only if for every z ε S , z ≠ x , y . Note that for a given set of nodes S the so-defined RN network is unique and does not depend on any subjectively imposed thresholds on the underlying distance structure. Mapping vector profiles on RN network Each accession is considered as a node, specified by its latitude and longitude. Moreover, to illustrate the method, we consider that each site (accession) x ε S is described by its metabolic profile over m metabolites. For the set of nodes, S , containing n given accessions, we first calculate the corresponding RN network based on the available geographic origin information. Given a geometric graph G , we then determine the weight θ xy of each edge ( x , y )ε E ( G ) as the Euclidean distance between the ( z -normalized) metabolic profiles of its incident nodes, that is, . In addition, each accession is characterized by the mean of the weights of its neighbours; in other words, an accession x is assigned a weight such that , where k ( x ) denotes the degree (number of neighbours) of the node x . Finally, the entire graph G is associated a weight . Any appropriate distance measure, as detailed above, can be used to map different types of profiles on the RN network. The local weights, establishing the connexion between the profiles of each accession and its immediate geographic neighbourhood, can further be subjected to the classical GV analysis, including the Moran’s I , Geary’s C and the Global G statistics [40] . Values for Moran’s I closer to 1 indicate positive, while values closer to −1 indicate negative spatial autocorrelation; a value of zero signifies random spatial pattern. The values for Geary’s C lie in the range between 0 and 2. Here a value of 1 indicates random spatial pattern, while values smaller (larger) than 1 indicate negative (positive) spatial autocorrelation. On the other hand, Global G seeks to establish if there are spatial bursts of high (low) values in an otherwise homogeneous space. To capture the effects of the sparse proximity structure in combination with climate factors, we also tested a spatial simultaneous autoregressive lag model for We used the five climate characteristics: air temperature, daily maximum air temperature, daily minimum air temperature, relative humidity, and daylight hours, as additional variables in the autoregressive model. The spatial autoregressive parameter ( rho ) was calculated with the trace approximation method [48] implemented in the Lagsarlm function from the spdep package in R [49] . Statistical sensitivity analysis In this section we detail the statistical sensitivity analysis, which can be used to determine the metabolites of highest influence to the outcome of GV analysis. The method relies on the proposed θ x statistic for each accession and Moran’s I statistic; it consists of the following steps: 1 Determine Moran’s I based on the θ x statistic over the entire metabolic profile, and call it I obs 2 For every metabolite M 3 Determine Moran’s I based on the θ x statistic calculated based on the metabolic profile from which the metabolite M is excluded 4 Assign the obtained value for I as a weight of the metabolite, and call it I M 5 End for 6 For every metabolite M 7 Calculate the difference Δ M = I obs − I M 8 End for 9 Perform a z -transformation on the obtained vector Δ 10 Report the metabolites whose z -score is at least half s.d. above/below the mean Robustness analysis The findings from the analysis of phenotypic and genetic variability with respect to geography may vary depending on the considered accessions. To establish a quantitative measure for the robustness of the findings from the analyses based on the dense (global), as well as the sparse (local) structure, we first calculated all statistics upon 100 random removals of 5, 10, 15, 20, and 25% of the analysed accessions. As the employed statistics take positive and negative values, we considered the squared coefficient of variation as a quantitative measure for comparison of the robustness from the different analyses and data types [50] . How to cite this article: Kleessen, S. et al . Structured patterns in geographic variability of metabolic phenotypes in Arabidopsis thaliana . Nat. Commun. 3:1319 doi: 10.1038/ncomms2333 (2012).